LEAFY COTYLEDON1 expression in the endosperm enables embryo maturation in Arabidopsis The endosperm provides nutrients and growth regulators to the embryo during seed development. LEAFY COTYLEDON1 (LEC1) has long been known to be essential for embryo maturation. LEC1 is expressed in both the embryo and the endosperm; however, the functional relevance of the endosperm-expressed LEC1 for seed development is unclear. Here, we provide genetic and transgenic evidence demonstrating that endosperm-expressed LEC1 is necessary and sufficient for embryo maturation. We show that endosperm-synthesized LEC1 is capable of orchestrating full seed maturation in the absence of embryo-expressed LEC1 . Inversely, without LEC1 expression in the endosperm, embryo development arrests even in the presence of functional LEC1 alleles in the embryo. We further reveal that LEC1 expression in the endosperm begins at the zygote stage and the LEC1 protein is then trafficked to the embryo to activate processes of seed maturation. Our findings thus establish a key role for endosperm in regulating embryo development. Seed development in angiosperm is a complex process that is initiated by the double fertilization of egg and central cells with two sperm cells that generate the diploid embryo and the triploid endosperm, respectively [1] . The endosperm plays an essential role in seed development by nourishing the embryo via transferring maternal nutrients and growth regulators [2] . The development of embryo and endosperm depends on both parental genomes and is influenced by the communication and coordination of their genetic programs [3] . Although progress has been made [2] , [4] , the molecular interactions between the endosperm and the embryo during seed development are generally not well understood. Many transcription factors have been shown to regulate seed development; one of them is a nuclear factor Y (NF-Y) transcription factor LEAFY COTYLEDON1 (LEC1) that has been identified as a key regulator of seed development [5] . In the embryo, LEC1 regulates seed development programs via combinatorial interactions with other transcription factors including the AFL B3 domain proteins, ABI3 , FUS3 , and LEC2 , which are all master regulators of seed maturation [5] , [6] , [7] , [8] , [9] , [10] . Null mutations in LEC1 cause defective seed phenotypes, including short embryo axis, less-developed cotyledons with anthocyanin accumulation, and desiccation intolerance [11] , [12] . Nonetheless, the lec1 homozygous plants rescued from mutant embryos did not exhibit any morphological abnormalities; neither were developmental paces and flowering time (Supplementary Fig. 1 ). As previously reported [5] , although there were no obvious morphological difference between wild type and the lec1-1 embryos from the globular to linear stages, embryos with purple cotyledons were observed from the lec1-1 mutant at early maturation (Supplementary Fig. 2 ). LEC1 expression has been detected not only in the embryo but also in the endosperm in several plant species, including Arabidopsis thaliana [13] , Brassica napus [14] , and soybean [10] , leading to speculation about a role of LEC1 in endosperm development [5] . However, no obvious morphological defects in the endosperm have been observed in lec1 mutant seeds [15] . We hypothesized that the endosperm-expressed LEC1 may act as a molecular signal in the early communication between endosperm and embryo, and subsequently exerts its key roles in activating and regulating various embryo developmental programs. In the following sessions, we present the results of our genetic and transgenic experiments designed to test this hypothesis. Expression of LEC1 in the endosperm is required for seed maturation To investigate if the expression of LEC1 in the endosperm was necessary for seed maturation, we generated seeds with unfertilized endosperms of lec1 genotype and fertilized diploid embryos of LEC1 genotype using a genomic imprinting bypassing strategy (Fig. 1a ), through which small but fully developed seeds could be produced when fis -class mutant flowers were crossed with cdka;1 mutant pollens [16] , [17] . We first generated two double mutant lines, fis2-6 +/− lec1-1 −/− and cdka;1 +/− lec1-1 −/− . In the self-crossed siliques of the double mutants, half of the seeds were arrested at early development stages, as was seen in the self-crossed fis2-6 +/− and cdka;1 +/− single mutants. The rest of the sibling seeds showed lec1 mutant phenotype as expected (Fig. 1b and Supplementary Fig. 3a ). To obtain seeds with lec1 endosperms and LEC1 embryos, we crossed fis2-6 +/− lec1-1 −/− flowers with cdka;1 +/− pollens (Fig. 1a ). Meanwhile, crosses of fis2-6 +/− × cdka;1 +/− and fis2-6 +/− × cdka;1 +/− lec1-1 −/− were also conducted as positive controls, and that of fis2-6 +/− lec1-1 −/− × cdka;1 +/− lec1-1 −/− as negative control (Supplementary Fig. 3b–d ). The F1 siliques had three types of seeds: normal size ( CDKA;1 +/+ ), small ( cdka;1 +/− ), and aborted (Fig. 1b–m ). The normal sized seeds and small seeds were classified as not aborted (NA) (Fig. 1c ) and they were distinguished by the size of seed area (normal seeds: above 0.15 mm 2 , small seeds: <0.1 mm 2 ) as reported previously [16] . Of note, genotype CDKA;1 +/+ represents the normal sized seeds (Fig. 1d–g ) which were wild type for both the FIS2 and CDKA;1 genes (maternal FIS2-6 + CDKA;1 + ; paternal FIS2-6 + CDKA;1 + ) since the maternal FIS2-6 + CDKA;1 + paternal FIS2-6 + cdka;1 − genotype seeds aborted at the pre-globular stage (Fig. 1m ). Genotype cdka;1 +/- represents the small seeds (Fig. 1h–k ) which were formed from maternal fis2-6 − CDKA;1 + and paternal FIS2-6 + cdka;1 − since the maternal fis2-6 − CDKA;1 + paternal FIS2-6 + CDKA;1 + genotype seeds aborted at the heart stage (Fig. 1l ). Further, the genotypes of the CDKA;1 +/+ and cdka;1 +/− seeds were confirmed by PCR-based genotyping at the CDKA;1 + /cdka;1 − and the LEC1 + /lec1 − loci in the seedlings derived from each type of seeds (Supplementary Fig. 3e ). Notably, the small seeds from the positive controls contained fully developed embryos (Fig. 1h, i ). The small seeds from the crosses of fis2-6 +/− lec1-1 −/− × cdka;1 +/− , with lec1 −/− endosperm and LEC1 +/− embryo, on the other hand, showed defective embryo phenotype (Fig. 1j ) that was also observed in the small seeds from the negative control, with lec1 −/− endosperm and lec1 −/− embryo (Fig. 1k ). Together, these results indicated that the expression of LEC1 in the endosperm was necessary for embryo maturation. Fig. 1: Loss-of-function of LEC1 in the endosperm disrupts seed development. a Cartoon showing a fis2-6 − lec1 − female gamete crossing with a cdka;1 − LEC1 + pollen to generate a small seed with lec1 −/− endosperm and LEC1 +/− embryo. Red dot, mutant lec1 − allele; black dot, wild type LEC1 + allele. Em embryo, Endo endosperm. b Green mature siliques collected from different genetic crosses. lec1 seeds display purple color. Arrows represent aborted seeds (red, fis2 − phenotype; black, cdka;1 − phenotype); asterisks indicate small seeds generated from the fis2-6 − × cdka;1 − bypassing cross. Five siliques from each of the five crosses were examined. Scale bar: 500 μm. c Percentage of various progeny produced from the bypassing genetic crosses. CDKA;1 +/+ indicate the normal sized wild type seeds, while cdka;1 +/− indicate the small seeds. NA not aborted seeds, A aborted seeds, n number of seeds scored. d – k Images of the CDKA;1 +/+ (normal size) and the cdka;1 +/− (small) seeds with different genotypes produced from the bypassing genetic crosses. Five seeds from each genotype were examined. The crosses of fis2-6 +/− × cdka;1 +/− produce d type normal seeds and h type small seeds. The crosses of fis2-6 +/− × cdka;1 +/ − lec1-1 −/ − produce e type normal seeds and i type small seeds. The crosses of fis2-6 +/ − lec1-1 −/− × cdka;1 +/− produce f type normal seeds and j type small seeds, while the crosses of fis2-6 +/ − lec1-1 −/− × cdka;1 +/ − lec1-1 −/− produce g type normal size lec1 seeds and k type small seeds. l An example of aborted seeds produced by fis2 - 6 − . Five seeds were examined. m An example of aborted seeds produced by cdka ; 1 − . Five seeds were examined. Scale bar: 100 μm. Full size image Haploid seeds with LEC1 endosperms and lec1 embryos develop normally To test whether the expression of LEC1 in the embryo was required for seed maturation, we generated seeds with haploid lec1 embryos and normal LEC1 endosperms by pollinating flowers of a haploid induction line (SeedGFP-HI), which was generated by introducing a transgene expressing an altered form of CENH3 fused with GFP and also a transgene expressing GFP driven by the seed storage protein gene At2S3 promoter in the cenh3-1 line [18] , [19] , with lec1-1 pollen grains (Fig. 2a ). We also conducted crosses of SeedGFP-HI flowers with wild type (WT) pollens to serve as control. From the SeedGFP-HI × lec1-1 and SeedGFP-HI × WT crosses, we harvested the mature siliques containing a mixture of haploids and hybrid diploids in addition to a high frequency of aborted seeds (Fig. 2b ). The diploid and haploid seeds were further hand-sorted based on their fluorescence patterns, as described previously [18] . The diploids with both embryo and endosperm inheriting the At2S3:GFP transgene in their maternal genome from the maternal parent SeedGFP-HI developed into seeds with uniform GFP signal, while the haploids with only the endosperm inheriting the maternal genome developed into seeds with mottled GFP fluorescence (Fig. 2c ). From the crosses of SeedGFP-HI × lec1-1 , haploid seeds with no lec1-1 seed defect (i.e., dark purple color) were obtained, which phenotypically resembled the haploid seeds from the SeedGFP-HI × WT crosses (Fig. 2c ). To examine the embryo phenotypes, we dissected the diploid and haploid seeds. We observed that both diploid and haploid seeds collected from the SeedGFP-HI × lec1-1 and the SeedGFP-HI × WT crosses contained fully developed embryos. The phenotypes of those diploid and haploid embryos highly resembled WT embryos and were clearly distinguishable from the lec1-1 embryos (Fig. 2d ). Diploid embryos were confirmed with the presence of GFP fluorescence and haploid embryos were GFP-negative (Fig. 2d ). Fig. 2: Fully developed haploid seeds with lec1 embryos and LEC1 endosperms. a Cartoon showing the genetic cross using the SeedGFP-HI line as female parent and lec1-1 as male parent to induce haploid progeny. Red dot: mutant lec1 − allele; black dot: wild type LEC1 + allele; green dot: weak centromeres CENH3-GFP from the HI parent; white dot: wild type centromeres. Em embryo, Endo endosperm. Note: the At2S3:GFP reporter in the SeedGFP-HI line is not shown in the cartoon. b Typical siliques containing GFP florescent seeds produced from the SeedGFP-HI × wild type (WT) or SeedGFP-HI × lec1-1 crosses. Approximately 30 siliques were produced from each type of the genetic crosses. Red arrows represent aborted seeds; black arrows indicate diploid seeds; white arrows indicate haploid seeds. Scale bar: 1000 μm. c Diploid and haploid seeds hand-sorted by their GFP signal patterns: seeds with uniform GFP signals (diploid) and seeds with mottled GFP fluorescence (haploid). At least four seeds from each genotype were examined for each replicate. This experiment was repeated three times independently. Scale bar: 500 μm. d Hand-dissected embryos from the mature diploid and haploid seeds produced from the crosses. Seed GFP florescence were detected under UV lights. Three embryos from each genotype were examined. Scale bar: 100 μm. e Detection of GFP signals in the centromere of root tip cells under confocal microscope. Insets: magnified areas of root cells indicated. Cell walls stained with propidium iodide (PI) are shown in red. Confocal images are shown as the merged channel of GFP and PI. Three embryos of each seed type were examined. This experiment was repeated three times independently. WT and lec1-1 embryos were used as control. Scale bar: 50 μm. Full size image The dissected diploids and haploids embryos were placed on MS agar plates to develop for subsequent genotype analysis. The diploid embryos were identifiable based on GFP signals observed at the centromeres in the root tip cells (Fig. 2e ), because they inherited the CENH3-GFP transgene from the HI line. The haploid embryos only inherited genome information from the paternal plant lec1-1 , thus displaying no GFP signal (Fig. 2e ). To further validate the identities of the diploids and haploids, we examined the morphology and genotype of the plants developed from the dissected embryos. In comparison with the diploid plants, the haploid plants showed reduced stature featuring narrower and smaller leaves (Supplementary Fig. 4a ), as previously observed [19] . During the reproductive phase, the diploid plants derived from the SeedGFP-HI × lec1-1 crosses produced normal size siliques that were filled with seeds segregating for the lec1-1 and wild type phenotypes (Supplementary Fig. 4b ). In contrast, the haploid plants from the same crosses produced only a few siliques with 1–2 seeds of the lec1-1 genotype. Similarly, haploid plants from the SeedGFP-HI × WT crosses produced siliques containing 1–2 seeds of the wild type genotype (Supplementary Fig. 4b ). To confirm that the haploids from the SeedGFP-HI × lec1-1 cross only inherited the genome from the lec1-1 paternal parent, we genotyped both the diploid and haploid plants derived from the cross at the LEC1 locus and detected both the wild type LEC1 allele and the lec1-1 T-DNA allele in the diploid plants but only the lec1-1 T-DNA allele in the haploid plants (Supplementary Fig. 4c ). These results further confirmed the identity of the haploid and the diploid seeds generated from the SeedGFP-HI × lec1-1 crosses. The facts that the presence of wild type LEC1 allele inherited from the maternal parent in the endosperm of haploids as evidenced by the mottled seed GFP signals and that the haploid seeds did not exhibit any lec1-1 defective seed phenotypes such as purple cotyledons and short embryo axis (Fig. 2c, d ) indicate that the seeds with LEC1 endosperm and lec1 embryo could develop normally through maturation. These results demonstrated that LEC1 gene expression in the embryo was dispensable for embryo maturation. Expressing LEC1 exclusively in the endosperm rescues the lec1 seed phenotype To further investigate whether an exclusive expression of LEC1 in the endosperm can rescue lec1 seed defects, we employed two endosperm-specific promoters, proPHERES1 ( pPHE ) [20] , [21] and proZHOUPI ( pZOU ) [22] , to direct the expression of LEC1 in lec1 mutants. We built two endosperm-specific expression constructs, pPHE::LEC1-GFP (PPL) and pZOU::LEC1-GFP (PZL), as well as controls that include pLEC1::LEC1-GFP (PLL), pPHE::ABI3-GFP (PPA), pZOU::ABI3-GFP (PZA), pPHE::GFP (PPg), and pZOU::GFP (PZg) (Supplementary Fig. 5 ). These constructs were introduced individually into embryo-rescued lec1-3 homozygous plants. From the T1 generation of PPL and PZL plants, 67% and 74% of the seeds (T2), respectively, were rescued to normal phenotype (Fig. 3a ). Among the lines introduced with the control constructs, 79% of the embryos from the PLL plants showed normal phenotype, but none were found in the PPA, PPg, and PZA lines (Fig. 3a ). We then tested the germination of T2 seeds to test if the transgenic seeds were desiccation-tolerant. As shown in Fig. 3b and Supplementary Fig. 6 , seeds from the PPL, PZL, and PLL lines germinated successfully, while those from PPA, PPg, and PZA succumbed to desiccation. Morphologically, the mature seeds of PPL, PZL, and PLL were indiscernible from that of wild type, but the PPA, PPg, and PZA seeds resembled that of lec1-3 (Fig. 3c–m ). The PPL, PZL, and PLL seeds possessed wild type levels of storage proteins (12S and 2S) while PPA, PPg, and PZA exhibited much lower levels similar to that of lec1-3 (Fig. 3n ). In addition, the same transgene constructs were also introduced into the lec1-1 plants in parallel and analogous results were obtained (Supplementary Fig. 7 ). Hence, LEC1 directed to be expressed solely in the endosperm was fully capable of complementing lec1 mutant seed in embryo morphology, seed germination, and storage protein accumulation. These transgenic experiments, in combination with the above described genetic evidence obtained from the haploid seed experiment, established that exclusive expression of LEC1 in the endosperm is sufficient to capacitate normal embryo development. Fig. 3: Gain-of-function of LEC1 in the endosperm rescues lec1-3 mutant seed phenotype. a Green mature siliques collected from T1 plants with different transgenes in the lec1-3 background. Siliques of T1 plants PLL-1 ( pLEC1::LEC1-GFP lec1-3 −/− ), PPL-1 ( pPHE::LEC1-GFP lec1-3 −/− ), and PZL-1 ( pZOU::LEC1-GFP lec1-3 −/− ) contain two types of seeds: [WT] seeds and [ lec1-3 ] seeds. PPA-1 ( pPHE::ABI3-GFP lec1-3 −/− ), PPg-1 ( pPHE::GFP lec1-3 −/− ), and PZA-1 ( pZOU::ABI3-GFP lec1-3 −/− ) only produce defective seeds ( lec1-3 ). [WT] indicates WT phenotype, [ lec1-3 ] indicates lec1-3 phenotype. At least five independent individual transgenic lines were examined for each construct transformation. Images of a typical embryo from each line are shown on the right next to the images of the siliques. WT (Ler-0) and lec1-3 are used as control. N normal seeds, A abnormal seeds ( lec1-3 ), n number of seeds scored. Em embryo. Scale bar: 500 μm. b Germination of seeds with different transgenic backgrounds at day 7. Fifty seeds were used for one biological germination test. This experiment was repeated three times independently. c – m Phenotypes of mature seeds from each of the transgenic backgrounds as indicated. Ten seeds from each genotype were examined. Scale bar: 300 μm. n SDS-PAGE gel image showing the 2S and 12S storage proteins in seeds from each of the transgenic backgrounds. This experiment was repeated three times independently. Full size image The onset of LEC1 expression occurs first in the endosperm To decipher the initiation and the mode of action of the endosperm-expressed LEC1 , we closely monitored GFP signals in the developing seeds of PLL, PPL, and PPg from the zygote stage onward, to maturation stage (Fig. 4a–u ). Pollen grains and ovules in the PLL before fertilization were also examined, and no GFP signal could be detected (Supplementary Fig. 8a, b ). GFP signals were first emerged from fertilized central cell (endosperm) nuclei in the PLL, PPL, and PPg seeds at the zygote stage (Fig. 4a–c and Supplementary Fig. 8c–e ). By the two-cell stage, GFP signals began to appear in the pro-embryo of PLL, in both the endosperm and the pro-embryo of PPL, but restricted to endosperm only in the PPg seeds (Fig. 4d–f and Supplementary Fig. 8f–h ). In the PLL embryos, GFP signals were observed from the globular to bent stages, but not at the maturation stage (Fig. 4g, j, m, p, s ). Similarly, the PPL embryos exhibited GFP signals at the globular, heart, linear, and bent stages, but not the maturation stage (Fig. 4h, k, n, q, t ). Notably, strong signals were present in the suspensors of PLL and PPL embryos (Fig. 4d, e, g, h, j, k ). Similar to observations from the PPL, GFP signals were also detected in developing embryos of the PZL seeds (Supplementary Fig. 8i, j ). In contrast, there was no GFP signal in the PPg embryos at any stages (Fig. 4c, f, i, l, o, r, u ). In the PPA seed, consistent with its lec1 mutant embryo phenotype, GFP signals were only detected in the endosperm nuclei at the pre-globular stage, but not in the embryos (Supplementary Fig. 9 ). Fig. 4: Endosperm-expressed LEC1 enters embryo to regulate seed maturation genes. a – u Localization patterns of GFP signals in PLL, PPL, and PPg seeds at various seed development stages from zygote to maturation as indicated. Five seeds or embryos at each stage from each line were examined. Embryos ( a – f ) are outlined in white dash lines for clarity. Amber stars indicate endosperm nuclei and white stars indicate embryo nuclei. GFP signals are shown in green. Cell walls stained with PI are shown in red. Shown here are merged confocal images from GFP and PI channels. Scale bars: 20 μm ( a – l ); 50 μm ( m – o ); 100 μm ( p – u ). v Relative expression of GFP in the whole seeds of PLL, PPL, PPg, and WT at linear stage. w Relative expression of GFP in the embryos (em) of PLL, PPL, PPg, and WT seeds at linear stage. x Relative expression of LEC2, FUS3 and ABI3 in the embryos (em) of PLL, PPL, PPg seeds at linear stage. v – x a to b indicate statistical difference with one-way ANOVA followed by the post-hoc Tukey multiple comparison tests ( p < 0.05). The CACS gene was used as an internal control. Values are mean ±  standard error of three biological replicates. Full size image To determine whether the LEC1 in the embryos of PPL was mobilized from the endosperm, we further generated a PPL-GFP 3 line expressing LEC1 fused to 3 copies of GFP (Supplementary Fig. 10a ). Such fusion proteins with multimeric GFPs have been employed successfully by others to restrict the mobility of mobile transcription factors [23] , [24] . LEC1-GFP 3 signals were observed in the endosperm nuclei at the pre-globular stage, but not in the embryos at the pre-globular, globular, heart, or linear stages (Supplementary Fig. 10b ). These results suggest that the LEC1 fusion protein was restricted to the endosperm in the PPL-GFP 3 seeds. Consistent with the lost mobility of LEC1-GFP 3 , the fusion gene failed to rescue the lec1-1 seed defects (Supplementary Fig. 10c ). In addition, we generated another control, the pAtML1::LEC1-GFP lec1-1 −/− (PML) line, employing the embryo-specific AtML1 promoter to drive the exclusive expression of LEC1 in the embryo [25] . As expected, expression of the LEC1-GFP fusion in the PML was only observed in the embryos, and it could successfully rescue the lec1-1 seed defects (Supplementary Fig. 11 ). This result is consistent with earlier observations that the lec1 mutant endosperms do not show any obvious defect [5] , and is also in line with our observations presented above (Supplementary Fig. 2 ). In light of the endosperm specificity of pPHE , these results signified that in the PPL seeds the endosperm-expressed LEC1-GFP was trafficked to the embryo from its expression origin, the endosperm, to enable embryo maturation. Such an scenario is further supported by our data from the PPL-GFP 3 line. These results show that LEC1 was mobilized from the endosperm to the embryo at very early stages of seed development. The LEC1 protein enters the embryo from the endosperm To investigate whether LEC1 was mobilized from the endosperm to the embryo in the form of RNA or protein, we performed RT-qPCR analyses to determine if there was any LEC1-GFP mRNA in the embryos. First, we measured the relative expression of GFP in the homozygous PLL, PPL, PPg, and WT (negative control) whole seeds at the linear stage, confirming the presence of GFP transcripts in the PLL, PPL, and PPg seeds (Fig. 4v ). We then measured the GFP mRNA in the linear stage embryos of PLL, PPL, using PPg and WT as negative controls since they had no GFP signal in the embryos. GFP mRNA was detected in the PLL embryos but not in the PPL embryos (Fig. 4w ). This result, when combined with the observation of clear presence of LEC1-GFP signals in the PPL embryos, strongly suggests that LEC1 was transported in the form of protein from the endosperm to the embryo. Such a notion is also consistent with our observation that there was no GFP signal in the PPL-GFP 3 embryos. We lastly examined the effectiveness of endosperm-synthesized LEC1 in activating embryo maturation genes known to be downstream target genes of LEC1 [5] , [26] , including the AFL B3 transcription factor genes ABI3 , FUS3 , and LEC2 . Through analyzing a set of LEC1 ChIP-seq data from a previous study [10] , we were able to verify the LEC1 occupancy on the promoters of LEC2 , FUS3 , ABI3 and LEC1 (Supplementary Fig. 12 ). We then measured the relative expression levels of LEC2 , FUS3 , and ABI3 in the linear stage embryos of PLL, PPL, and PPg. As shown in Fig. 4x , similar levels of LEC2 , FUS3 , and ABI3 expression was detected in the PPL and PLL embryos, but almost negligible in the PPg embryos. These results demonstrated that the LEC1 protein synthesized in the endosperm adequately activates the seed development programs including the maturation genes without de novo LEC1 synthesis in the PPL embryo. Our study uncovers a mode of action of LEC1 that is initially expressed in the endosperm but subsequently in the form of LEC1 protein mobilized to the embryo as a molecular signal (Fig. 5 ). Given the LEC1-GFP strong signals being detected in the suspensors, we conjecture that the route of trafficking is via the suspensor, which has long been suspected of mediating symplastic transfer of metabolites and proteins from the endosperm to embryo [2] . The endosperm-synthesized LEC1 protein, once transported into the embryo, can subsequently trigger the expression of LEC1 in the embryo and ultimately the LEC1 -regulatory network to enable normal seed development. Such an scenario is also consistent with the postulated activity of LEC1 as a pioneer transcription factor [27] and the notion that the chromatin environment in the endosperm is distinct from that in the embryo [3] . Seed genes, particularly those pertinent to seed maturation, are believed to be repressed during vegetative growth by the polycomb proteins-mediated chromatin condensation [28] , [29] , [30] . How they get reset during seed development has been a puzzling question. Our findings provide a plausible explanation for the reprograming of these genes in the new generation (i.e., seed). It is conceivable that, due to the favorable chromatin and cellular environments in the endosperm, LEC1 becomes activated there shortly after fertilization and enters the embryo, where it overcomes the repressive chromatin context to trigger the de-repression of seed genes including itself. Fig. 5: A model depicting the regulation of seed maturation by the mobile transcription factor LEC1. In early stages of seed development, the onset of LEC1 expression occurs in the endosperm, followed by mobilization of the LEC1 protein to the embryo, likely via the plasmodesmata (PD) in the suspensor cells. After entering the embryo, the endosperm-synthesized LEC1 overcomes the repressive chromatin constraints to trigger the de-repression of seed maturation-related transcription factor genes including LEC2 , ABI3 , FUS3 , and LEC1 itself ( L.A.F.L . ). Subsequently, the L.A.F.L. transcription factors activate the expression of seed storage reserve synthesis genes, enabling normal seed maturation. In the lec1 mutant seeds, the L.A.F.L . network remains repressed due to lack of LEC1 expression in both the endosperm and the embryo, thus leading to dramatically reduced accumulation of seed storage reserves and consequently the formation of desiccation-intolerant purple seeds. Notes: endosperm (Endo), embryo (Em), and suspensor (Sp) are colored with light amber, light green, and light blue, respectively; amber circles represent endosperm nuclei; dark green circles indicate embryo nuclei; orange and gray circles represent wild type and mutant LEC1 proteins, respectively; black lines represent genomic DNA and the orange/black rectangular bars indicate the wild type and mutant LEC1 genes, respectively; purple circles represent histones; red stars represent repressive histone modifications, such as H3K27me3; and bright green squares represent seed storage reserves (SSPs: seed storage proteins). Full size image Why would a functional LEC1 copy remain expressed in the embryo, given that its expression in the endosperm seems to be enough to ensure proper seed development? It would be tempting to speculate that one advantage would be to have more-than-enough LEC1, as an enhanced mechanism, to enable/double-secure the normal embryo development, a vital process for a plant’s survival. Another puzzling question is why LEC1 expression in the embryo is normally dependent on LEC1 protein provided to the embryo by the endosperm. We would speculate that such an arrangement allows a spatial separation of the embryo and its key regulator, thus adding a new layer of control in the regulation of embryo development. This would make sure that embryo development, in particular the maturation program, would not initiate until it is informed to do so, i.e., after successful fertilization, otherwise remains securely repressed during the rest of the plant’s life cycle. In conclusion, we demonstrate the critical importance of endosperm-synthesized LEC1 in enabling normal seed development including maturation in Arabidopsis . These findings establish LEC1 as a molecular signal in the communication between the embryo and the endosperm during seed development, and thus provide novel insights into the mechanisms by which the endosperm nourishes and regulates embryo development. Plant materials and growth conditions Arabidopsis thaliana ecotypes Columbia-0 (Col-0) and Landsberg (Ler-0) were used as wild types. Arabidopsis mutant lines lec1-1 (SALK_131219) [27] , lec1-2 (CS870475), lec1-3 (CS5739) [31] , cdka;1 (SALK_106809.34.90.X) [16] , [17] , and fis2-6 (CS6998) were obtained from the Arabidopsis Biological Resource Center (ABRC). Haploid Inducer SeedGFP-HI line was a gift from UC Davis [18] , [19] . Transgenic plants of pLEC1::LEC1-GFP lec1 (PLL), pPHE::LEC1-GFP lec1 (PPL), pPHE::GFP lec1 (PPg), pPHE::ABI3-GFP lec1 (PPA), pZOU::LEC1-GFP lec1 (PZL), pZOU::GFP lec1 (PZg), pZOU::ABI3-GFP lec1 (PZA), pPHE::LEC1-GFP-GFP-GFP lec1 (PPL-GFP 3 ), and pAtML1::LEC1-GFP lec1 (PML) were generated in this work. Note: lec1 can be either lec1-1 or lec1-3 , as specified in the main text. Double mutant lines lec1-1 cdka;1 and lec1-1 fis2-6 were produced by genetic crosses. The wild type and mutant seeds were germinated either in soil or on half-strength MS medium and grown in a growth room with humidity of 65% under a 16 h light/8 h dark cycle at 22 °C. All genotypes were determined by PCR, by resistance to hygromycin, or by phenotype. 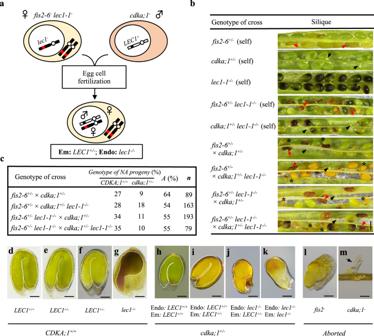Fig. 1: Loss-of-function ofLEC1in the endosperm disrupts seed development. aCartoon showing afis2-6−lec1−female gamete crossing witha cdka;1−LEC1+pollen to generate a small seed withlec1−/−endosperm andLEC1+/−embryo. Red dot, mutantlec1−allele; black dot, wild typeLEC1+allele. Em embryo, Endo endosperm.bGreen mature siliques collected from different genetic crosses.lec1seeds display purple color. Arrows represent aborted seeds (red,fis2−phenotype; black,cdka;1−phenotype); asterisks indicate small seeds generated from thefis2-6−×cdka;1−bypassing cross. Five siliques from each of the five crosses were examined. Scale bar: 500 μm.cPercentage of various progeny produced from the bypassing genetic crosses.CDKA;1+/+indicate the normal sized wild type seeds, whilecdka;1+/−indicate the small seeds. NA not aborted seeds, A aborted seeds, n number of seeds scored.d–kImages of theCDKA;1+/+(normal size) and thecdka;1+/−(small) seeds with different genotypes produced from the bypassing genetic crosses. Five seeds from each genotype were examined. The crosses offis2-6+/−×cdka;1+/−producedtype normal seeds andhtype small seeds. The crosses offis2-6+/−×cdka;1+/−lec1-1−/−produceetype normal seeds anditype small seeds. The crosses offis2-6+/−lec1-1−/−×cdka;1+/−produceftype normal seeds andjtype small seeds, while the crosses offis2-6+/−lec1-1−/−× cdka;1+/−lec1-1−/−producegtype normal sizelec1seeds andktype small seeds.lAn example of aborted seeds produced byfis2-6−. Five seeds were examined.mAn example of aborted seeds produced bycdka;1−. Five seeds were examined. Scale bar: 100 μm. Primers used for genotyping are listed in Supplementary Table 1 . Plasmid construction To generate the pLEC1::LEC1-GFP construct, the LEC1 genomic region from 2000 bp upstream of the ATG to the end of ORF without stop codon was amplified from Col-0 genomic DNA with primers F-pro-LEC1/R-LEC1 , transferred into pMDC107 [32] . To generate the pPHE::LEC1-GFP construct, the LEC1 genomic region from ATG to the end of ORF without stop codon was amplified from Col-0 genomic DNA with primers F-LEC1/R-LEC , ligated into pMDC107 to get the LEC1-GFP construct. Then the PHE promoter region (2000 bp upstream of the ATG) was amplified from Col-0 DNA with primers F-pro-PHE/R-pro-PHE , transferred to the LEC1-GFP construct. To build the pPHE::LEC1-GFP-GFP-GFP construct, GFP-GFP was amplified with primers Pme1-Mlu1-GFP-F / Asc1-GFP-R , transferred to pMDC107 to get the GFP-GFP-GFP construct. Then pPHE1::LEC1 was cloned with primers F-pro-PHE / Mlu1-LEC1-R , then transferred to the GFP-GFP-GFP construct. Similarly, to get the construct pPHE::ABI3-GFP , the ABI3 genomic region from ATG to the end of ORF without stop codon was amplified from Col-0 genomic DNA with primers F-ABI3/R-ABI3 , then ligated into pMDC107 to get the ABI3-GFP construct before introducing the PHE promoter amplified previously. To get the pPHE::GFP construct, the PHE promoter region (2000 bp upstream of the ATG) was amplified from Col-0 DNA with primers F-pro-PHE/R-pro-PHE-1 , ligated into pMDC107. To generate the pZOU::LEC1-GFP construct, the ZOU promoter region (2000 bp upstream of the ATG) was amplified from Col-0 DNA with primers F-pro-ZOU/R-pro-ZOU , then ligated to the LEC1-GFP construct. To get the construct pZOU::ABI3-GFP , the ZOU promoter amplified previously was cloned into ABI3-GFP . To get the pZOU::GFP construct, the ZOU promoter region (2000 bp upstream of the ATG) was amplified from Col-0 DNA with primers F-pro-ZOU/R-pro-ZOU-1 , ligated into pMDC107. To generate the pAtML1::LEC1-GFP construct, the AtML1 promoter region [25] was amplified from Col-0 DNA with primers pAtML1-F/pAtML1-R , then ligated to the LEC1-GFP construct. 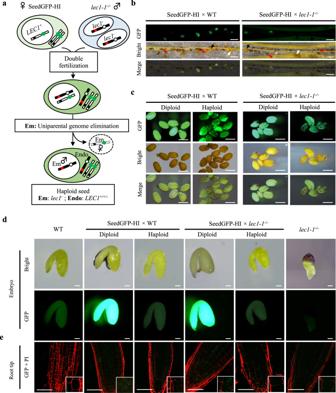Fig. 2: Fully developed haploid seeds withlec1embryos andLEC1endosperms. aCartoon showing the genetic cross using the SeedGFP-HI line as female parent andlec1-1as male parent to induce haploid progeny. Red dot: mutantlec1−allele; black dot: wild typeLEC1+allele; green dot: weak centromeres CENH3-GFP from the HI parent; white dot: wild type centromeres. Em embryo, Endo endosperm. Note: theAt2S3:GFPreporter in the SeedGFP-HI line is not shown in the cartoon.bTypical siliques containing GFP florescent seeds produced from the SeedGFP-HI×wild type (WT) or SeedGFP-HI× lec1-1crosses. Approximately 30 siliques were produced from each type of the genetic crosses. Red arrows represent aborted seeds; black arrows indicate diploid seeds; white arrows indicate haploid seeds. Scale bar: 1000 μm.cDiploid and haploid seeds hand-sorted by their GFP signal patterns: seeds with uniform GFP signals (diploid) and seeds with mottled GFP fluorescence (haploid). At least four seeds from each genotype were examined for each replicate. This experiment was repeated three times independently. Scale bar: 500 μm.dHand-dissected embryos from the mature diploid and haploid seeds produced from the crosses. Seed GFP florescence were detected under UV lights. Three embryos from each genotype were examined. Scale bar: 100 μm.eDetection of GFP signals in the centromere of root tip cells under confocal microscope. Insets: magnified areas of root cells indicated. Cell walls stained with propidium iodide (PI) are shown in red. Confocal images are shown as the merged channel of GFP and PI. Three embryos of each seed type were examined. This experiment was repeated three times independently. WT andlec1-1embryos were used as control. Scale bar: 50 μm. At least five independent transgenic lines for each construct transformation were obtained and examined. Primer information is listed in Supplementary Table 1 . Plant transformation was performed via floral dipping [33] . Seed rescue Immature siliques from lec1 heterozygous parental plants were collected and surface sterilized with 70% ethanol, dissected under a dissecting microscope. Homozygous mutant seeds (purple color, with defective embryos) were transferred to half-strength MS agar plates with 1% sucrose for germination. After germination, seedlings were then transferred to soil for further experiments. lec1 homozygosity was normally confirmed by PCR-based genotyping. Genetic crosses for the fis2-cdka;1 bypassing assay and haploid seed production To obtain the lec1 - 1 −/− fis2-6 +/− line, the lec1 - 1 homozygous mutant and fis2-6 heterozygous mutant plants were used for cross. The lec1-1 −/− flowers at stage 12 were emasculated and shortly after that the pistils were hand-pollinated with pollen grains from the fis2-6 +/− plants. F1 seeds from the cross were collected and planted to produce F2 seeds. The lec1 - 1 −/− fis2-6 +/− plants were selected based on the combination of phenotypes of lec1 - 1 −/− (purple color, not fully developed embryos) and fis2-6 +/− (aborted seeds at heart stage) from the F2 self-crossed siliques. Similarly, the lec1 - 1 −/− cdka;1 +/− line was obtained by crossing the lec1 - 1 −/− line and the cdka;1 +/− line. The cdka;1 +/− flowers at stage 12 were emasculated and the pistils were hand-pollinated with pollen grains from the lec1 - 1 −/− plants. F1 seeds from the crossed siliques were used to produce F2 seeds. The lec1 - 1 −/− cdka;1 +/− plants were confirmed by the combination of phenotypes of lec1 - 1 −/− (purple color, not fully developed embryo) and cdka;1 +/− (half amount of seeds aborted at heart stage in one silique) from the F2 self-crossed siliques. For FIS-CDKA bypassing assays, fis2-6 +/− and lec1 -1 −/− fis2-6 +/− lines were used as maternal parents while cdka;1 +/− and lec1 - 1 −/− cdka;1 +/− plants were used as pollen donor. For SeedGFP-HI experiments, the SeedGFP-HI flowers were emasculated at stage 12 and hand-pollinated with pollen grains from the lec1 - 1 −/− plants. Seeds were collected from the F1 siliques for further experiments. Microscopy For examination of seed morphology, siliques were hand-dissected for differential interference contrast (DIC) imaging by using a stereomicroscope. For examination of embryo development, seeds were mounted in the Hoyer’s solution for DIC [34] . The GFP florescence of seeds and embryos produced from the HI crosses were examined under UV lights with a stereomicroscope. The stereomicroscope used for the experiments was a Nikon SM225 equipped with a DS-Ri2 camera (Nikon). Confocal images were taken using an Olympus Fluoview FV1200 laser scanning microscope with excitation wavelength of 488 nm for EGFP and 559 nm for propidium iodide (PI). Confocal images were analyzed using the imaging software: OLYMPUS FLUOVIEW Ver.4.2. RT-qPCR analysis For RNA isolation, linear embryos were dissected as described previously with some modifications [35] . More specifically, individual embryos were hand-dissected under a stereomicroscope (EMZ PLS-2 stand, MEIJI) from seeds immersed in 10% RNAlater (Thermo Fisher Scientific) with fine point tweezers, and transferred with a 2–20 µl RNAse-free pipette tip (VWR) to depression slides (VWR) containing 200 µl of 10% RNAlater. After every 10 embryos dissected, the embryos were washed with 10% RNAlater three times, then transferred to 30 µl of 100% RNAlater. RNA was isolated from each pool of 50 embryos per sample by adding 500 µl TRIzol (Thermo Fisher Scientific) followed by incubation at 60 °C for 30 min, and then purified according to the TRIzol reagent protocol for RNA isolation from small quantities of tissue (Life Technologies). For each sample, 100 ng of RNA was used in reverse transcription reactions using a iScript Reverse Transcription Supermix for RT-qPCR kit (Bio-RAD). 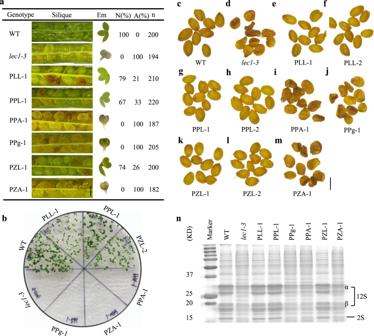Fig. 3: Gain-of-function ofLEC1in the endosperm rescueslec1-3mutant seed phenotype. aGreen mature siliques collected from T1 plants with different transgenes in thelec1-3background. Siliques of T1 plants PLL-1 (pLEC1::LEC1-GFP lec1-3−/−), PPL-1 (pPHE::LEC1-GFP lec1-3−/−), and PZL-1 (pZOU::LEC1-GFP lec1-3−/−) contain two types of seeds: [WT] seeds and [lec1-3] seeds. PPA-1 (pPHE::ABI3-GFP lec1-3−/−), PPg-1 (pPHE::GFP lec1-3−/−), and PZA-1 (pZOU::ABI3-GFP lec1-3−/−) only produce defective seeds (lec1-3). [WT] indicates WT phenotype, [lec1-3] indicateslec1-3phenotype. At least five independent individual transgenic lines were examined for each construct transformation. Images of a typical embryo from each line are shown on the right next to the images of the siliques. WT (Ler-0) andlec1-3are used as control. N normal seeds, A abnormal seeds (lec1-3), n number of seeds scored. Em embryo. Scale bar: 500 μm.bGermination of seeds with different transgenic backgrounds at day 7. Fifty seeds were used for one biological germination test. This experiment was repeated three times independently.c–mPhenotypes of mature seeds from each of the transgenic backgrounds as indicated. Ten seeds from each genotype were examined. Scale bar: 300 μm.nSDS-PAGE gel image showing the 2S and 12S storage proteins in seeds from each of the transgenic backgrounds. This experiment was repeated three times independently. For each quantification-PCR (qPCR), SsoFast EvaGreen Supermix (Bio-RAD) with Gene-specific and CACS (endogenous control) [36] primers were used to conduct qPCR reactions on a Bio-RAD C1000 TM Thermal Cycler with the CFX96 TM Real-time PCR System (Bio-RAD). qPCR data was analyzed using Bio-Rad CFX Manager program. Primer information is listed in Supplementary Table 1 . 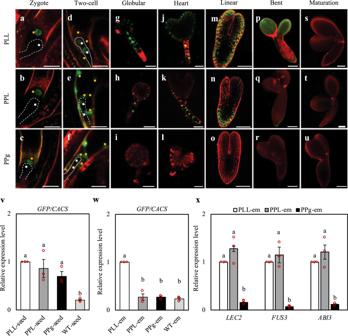Fig. 4: Endosperm-expressed LEC1 enters embryo to regulate seed maturation genes. a–uLocalization patterns of GFP signals in PLL, PPL, and PPg seeds at various seed development stages from zygote to maturation as indicated. Five seeds or embryos at each stage from each line were examined. Embryos (a–f) are outlined in white dash lines for clarity. Amber stars indicate endosperm nuclei and white stars indicate embryo nuclei. GFP signals are shown in green. Cell walls stained with PI are shown in red. Shown here are merged confocal images from GFP and PI channels. Scale bars: 20 μm (a–l); 50 μm (m–o); 100 μm (p–u).vRelative expression ofGFPin the whole seeds of PLL, PPL, PPg, and WT at linear stage.wRelative expression ofGFPin the embryos (em) of PLL, PPL, PPg, and WT seeds at linear stage.xRelative expression ofLEC2, FUS3andABI3in the embryos (em) of PLL, PPL, PPg seeds at linear stage.v–xa to b indicate statistical difference with one-way ANOVA followed by the post-hoc Tukey multiple comparison tests (p< 0.05). TheCACSgene was used as an internal control. Values are mean ±  standard error of three biological replicates. 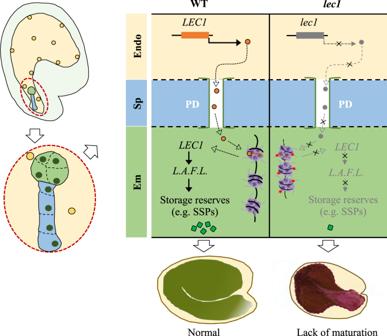Fig. 5: A model depicting the regulation of seed maturation by the mobile transcription factor LEC1. In early stages of seed development, the onset ofLEC1expression occurs in the endosperm, followed by mobilization of the LEC1 protein to the embryo, likely via the plasmodesmata (PD) in the suspensor cells. After entering the embryo, the endosperm-synthesized LEC1 overcomes the repressive chromatin constraints to trigger the de-repression of seed maturation-related transcription factor genes includingLEC2,ABI3,FUS3, andLEC1itself (L.A.F.L.). Subsequently, the L.A.F.L. transcription factors activate the expression of seed storage reserve synthesis genes, enabling normal seed maturation. In thelec1mutant seeds, theL.A.F.L. network remains repressed due to lack ofLEC1expression in both the endosperm and the embryo, thus leading to dramatically reduced accumulation of seed storage reserves and consequently the formation of desiccation-intolerant purple seeds. Notes: endosperm (Endo), embryo (Em), and suspensor (Sp) are colored with light amber, light green, and light blue, respectively; amber circles represent endosperm nuclei; dark green circles indicate embryo nuclei; orange and gray circles represent wild type and mutant LEC1 proteins, respectively; black lines represent genomic DNA and the orange/black rectangular bars indicate the wild type and mutantLEC1genes, respectively; purple circles represent histones; red stars represent repressive histone modifications, such as H3K27me3; and bright green squares represent seed storage reserves (SSPs: seed storage proteins). Storage protein analysis Mature seeds were ground in the extraction buffer (100 mM Tris-HCl pH 8.0, 1% SDS, 10% glycerol, and 2% β-mercaptoethanol). The extracts were boiled for 3 min, followed by centrifugation at 20,000 g for 5 min. The supernatant of each sample was transferred to a new tube. Protein samples were mixed with 5× loading buffer, denatured by adding 18.5 mM dithiothreitol, before loading onto 15% SDS-PAGE gels. After separation by electrophoresis using a Biochrom Novaspec Plus Visible Spectrophotometer (Bio-RAD), the protein gels were stained with Coomassie Brilliant Blue R250 for 30 min, followed by de-staining for 1 h with de-staining solution (10% glacial acid, 40% methanol) before imaging with a GS-900 Calibrated Densitometer scanner. Statistical analysis R v.3.6.3 ( http://www.r-project.org/ ) was used for the statistical analyses. Bartlett tests were performed to verify the equality of the variance across the samples. One-way ANNOVA analyses and post-hoc Tukey tests were conducted to determine the significant difference. Bar graphs were generated by using Microsoft Excel 2016. Reporting summary Further information on research design is available in the Nature Research Reporting Summary linked to this article.